Observation of atomic speckle and Hanbury Brown–Twiss correlations in guided matter waves Speckle patterns produced by multiple independent light sources are a manifestation of the coherence of the light field. Second-order correlations exhibited in phenomena such as photon bunching, termed the Hanbury Brown–Twiss effect, are a measure of quantum coherence. Here we observe for the first time atomic speckle produced by atoms transmitted through an optical waveguide, and link this to second-order correlations of the atomic arrival times. We show that multimode matter-wave guiding, which is directly analogous to multimode light guiding in optical fibres, produces a speckled transverse intensity pattern and atom bunching, whereas single-mode guiding of atoms that are output-coupled from a Bose–Einstein condensate yields a smooth intensity profile and a second-order correlation value of unity. Both first- and second-order coherence are important for applications requiring a fully coherent atomic source, such as squeezed-atom interferometry. Optical speckle is a textbook phenomena [1] that arises from interference between multiple wavefronts originating from independent sources, such as the microscopic features of a diffuse scattering material illuminated by a laser. In this case, the original light source (the laser) is coherent, and the multiple scattering sources therefore have a fixed phase relationship so that the speckle pattern does not vary in time. However, for an incoherent light source such as a distant star, the multiple independent sources on the disc of the star have fluctuating phases, yielding a temporally varying speckle intensity pattern [2] . The HBT effect was first observed using an incoherent laboratory light source [3] but was then applied to measure the optical spatial properties of stars [4] . The technique involved measuring the statistical distribution of arrival times τ between photon pairs, known as the second-order temporal correlation function g (2) ( τ ) normalized by the light intensity [4] . For incoherent sources of bosons (such as photons and bosonic atoms), particle bunching is expected, that is, there is an enhanced probability of multiple particles arriving within an interval that defines the coherence time of the source. In this case, the peak value of g (2) ( τ ) is enhanced by a factor of two, compared with the asymptotic value of unity for large arrival delay times. This temporal bunching can also be described in terms of the speckle pattern produced by multiple independent sources, the phases of which fluctuate [2] . Conversely, a highly coherent source such as an optical laser, a Bose–Einstein condensate (BEC) or an atom laser will exhibit a uniform arrival time probability for particle pairs, that is, no bunching. This yields a g (2) ( τ ) of unity for all delays, indicating long-range coherence [5] . Pioneering quantum statistical experiments undertaken elsewhere have measured second-order correlation functions for atoms in an analogue of the HBT experiment, demonstrating bunching for incoherent (thermal) sources of bosonic Ne* atoms [6] and 4 He* atoms [7] . Antibunching was also observed for fermionic 3 He *atoms [8] in a manifestation of the Pauli exclusion principle. In our laboratory, we have performed the first simultaneous measurement of the higher-order correlation functions g (2) ( τ ) and g (3) ( τ 1 , τ 2 ), using both thermal and Bose-condensed atoms [9] . However, in all of the above experiments, the sources were either completely coherent (in the case of a BEC) and therefore would not be expected to yield a speckle pattern, or were the result of a large number of poorly resolved sources such that the atomic density pattern would not reveal structure. Only in the case of a relatively small number of interfering matter-wave modes is speckle measurable using a detector with limited spatial resolution [5] . In the present experiments, we have resolved atomic speckle for the first time by using an atomic waveguide to limit the number of modes present. This is analogous to an optical fibre in which more than one mode is present, which thereby produces a speckled transverse light-intensity pattern. From a practical standpoint, atom guiding is an important technique in atom optics for transmitting atoms over macroscopic distances [10] , [11] , [12] , [13] , [14] , [15] , [16] , [17] , [18] , [19] , [20] , and in many applications, knowledge of the coherence of the matter-wave transmission is an important requirement. We not only measure directly the speckle properties of the guided matter waves, but we also relate this to the second-order correlation function g (2) ( τ ) to demonstrate that speckle is characterized by atom bunching. Experiment overview In our experiments, we guide He* atoms that are in a long-lived metastable state [21] possessing ∼ 20 eV of internal energy and allowing single atom detection. A single 1,550-nm focused laser beam provides the guiding potential, which minimizes spontaneous scattering of photons because of its large red detuning from the relevant He* transition (1,083 nm). However, the dipole force exerted by the laser beam is significant and enables the confinement of He* atoms. The beam is focussed vertically with a maximum power of 60 mW (equating to a trap depth of ∼ 7 μK) and creates a trap at high power, which can be transformed into a waveguide at lower power. 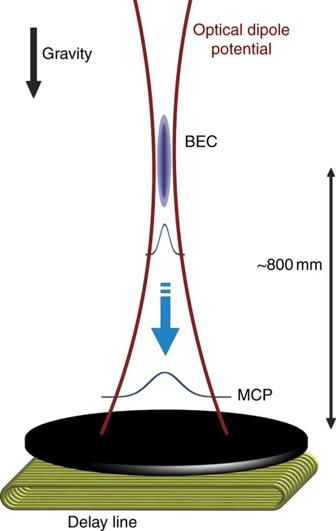Figure 1: Experimental schematic. A thermal cloud/Bose–Einstein condensate (BEC) is confined in an optical trap, produced by a single focused laser beam in the vertical direction. By reducing the power in the optical beam, the cloud is no longer supported against gravity and falls towards the single-atom microchannel plate (MCP) detector. The transverse potential is still strong enough to confine the atoms in that direction so the atoms are effectively guided. The basic experimental setup is shown in Figure 1 . Figure 1: Experimental schematic. A thermal cloud/Bose–Einstein condensate (BEC) is confined in an optical trap, produced by a single focused laser beam in the vertical direction. By reducing the power in the optical beam, the cloud is no longer supported against gravity and falls towards the single-atom microchannel plate (MCP) detector. The transverse potential is still strong enough to confine the atoms in that direction so the atoms are effectively guided. Full size image Experimental procedure To prepare atoms in the guide, He* atoms are initially pre-cooled to just above the BEC transition temperature, T c , in a BiQUIC magnetic trap [22] before being transferred into the dipole potential, at which a condensate fraction is formed. To release atoms into the guide, the laser intensity is reduced until the atoms are no longer held against gravity in the weak axis of the trap, at which point they fall and are guided by the transverse confinement of the dipole potential. Spatial speckle experiments By tuning the laser intensity at which we guide atoms and the initial temperature before guiding, we can guide either ultracold thermal (incoherent) or Bose-condensed (coherent) atoms. For single-mode guiding, we evaporate nearly all of the thermal atoms to create as pure a condensate as possible and then transfer the condensate adiabatically from the trap to the guide to minimize excitations. Near single-mode guiding of a condensate with 65% of atoms occupying the lowest mode [20] has been demonstrated using these techniques. The production of multimode beams is made more complicated by the BEC, which is always present because of our transfer procedure from the magnetic to the optical trap. Multimode beams can still be created, however, by reducing the trapping potential to a point at which thermal atoms can escape from the trap, whereas the colder BEC still remains trapped. The different source-loading procedures therefore lead to guide potentials that are slightly different for single or multimode guiding. Our initial experiments were performed by guiding ∼ 10 5 He* atoms onto a microchannel plate (MCP) and phosphor screen detector, located ∼ 180 mm below the trap. Here we transfer only thermal atoms into the guide, and the resulting detector image displays matter-wave speckle (see Fig. 2a–c ). By averaging the intensity over 20 runs of the experiment ( Fig. 2d ), the speckle washes out confirming that it is indeed due to the interference of many modes in the guide with random phases. 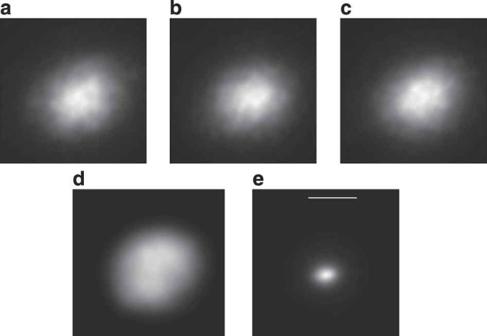Figure 2: Multimode speckle images. (a–c) Successive experimental realizations produced by guiding only the thermal component of the trapped atoms, showing interference between the thermal modes ('speckle'). Each panel (a–c) is a single experimental run, and the pattern is seen to change between images because of the random nature of the speckle for different realizations of the experiment. (d) Average of 20 runs of the experiment, (e) image of a predominantly single-mode profile. All five images show a 3×3 mm2window. Scale bar, 1 mm. For comparison, an image of a single-mode guided spot is shown in Figure 2e , which has a smaller radius and a cleaner Gaussian profile with no speckle visible. Figure 2: Multimode speckle images. ( a – c ) Successive experimental realizations produced by guiding only the thermal component of the trapped atoms, showing interference between the thermal modes ('speckle'). Each panel ( a – c ) is a single experimental run, and the pattern is seen to change between images because of the random nature of the speckle for different realizations of the experiment. ( d ) Average of 20 runs of the experiment, ( e ) image of a predominantly single-mode profile. All five images show a 3×3 mm 2 window. Scale bar, 1 mm. Full size image Hanbury Brown–Twiss guiding experiments The idea that matter-wave speckle, as observed in our experiments, is a direct demonstration of the HBT effect is intriguing. To investigate this analogy, we use a MCP and delay line detector located 848 mm below the trap (see Fig. 1 ) to allow true single-atom counting correlation experiments to be performed [23] . 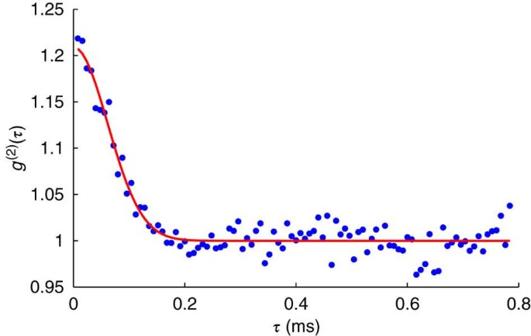Figure 3: Bunching of a multimode cloud. Temporal second-order correlation function of a guided multimode thermal cloud. Blue circles are the experimental points, whereas the red line shows a fit with a gaussian correlation function. Figure 3 shows the significant bunching signal observed in the temporal second-order correlation function of a guided thermal cloud of atoms. The measured bunching amplitude of g (2) (0)=1.21 is the largest bunching signal ever observed with atoms, more than three times larger than the previous highest signal [7] . The large bunching amplitude is due to the low effective transverse temperature ( ∼ nK) and large correlation lengths occurring within the guide, which prevents the signal from washing out because of imperfect detector resolution. Note that the noise present in Figure 3 is predominantly shot noise. Thus, for large time separations τ , at which the number of pairs decreases, there is an associated increase in the spread of g (2) . Figure 3: Bunching of a multimode cloud. Temporal second-order correlation function of a guided multimode thermal cloud. Blue circles are the experimental points, whereas the red line shows a fit with a gaussian correlation function. Full size image Bunching amplitude for different mode occupancies To investigate quantitatively the variation of bunching amplitude with transverse mode occupancy, we load thermal clouds of different temperatures into the guide and determine the two-particle correlation function as calculated previously [23] . 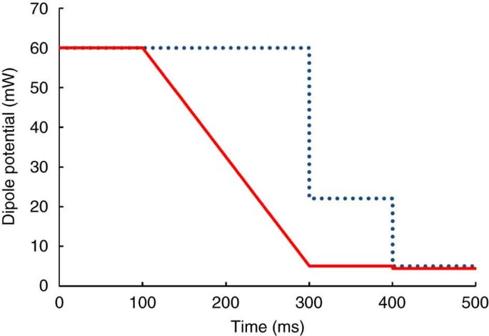Figure 4: Timing diagram for guiding experiments. The procedures for loading a single-mode (BEC) or a multimode (thermal gas) into the guide are shown as a solid red line and a dashed blue line, respectively. The energy of the thermal clouds loaded into the guide is set by the depth of the truncation cut, shown at 300 ms. The procedure for loading different thermal distributions (and thus different transverse mode occupancies) is shown diagrammatically in Figure 4 . After transferring atoms into the optical trap, we rapidly reduce the trap depth to evaporate the hotter atoms in the distribution. The depth of this cut in the trap depth determines the thermal energy of the remaining atoms and thereby allows us to control the number of transverse modes excited in the guide. A 100-ms period of thermalization then follows to ensure that the thermal equilibrium is established. To transfer atoms into the guide, the trap potential is stepped down to the final guiding potential, which is the same value for all our multimode guiding experiments. Figure 4: Timing diagram for guiding experiments. The procedures for loading a single-mode (BEC) or a multimode (thermal gas) into the guide are shown as a solid red line and a dashed blue line, respectively. The energy of the thermal clouds loaded into the guide is set by the depth of the truncation cut, shown at 300 ms. Full size image The spatial distribution at the detector is used to determine the relative mode occupancy by fitting the measured profile with a linear superposition of transverse modes for a harmonic potential. The relative populations in each mode are then combined to yield an average transverse mode occupancy [18] . 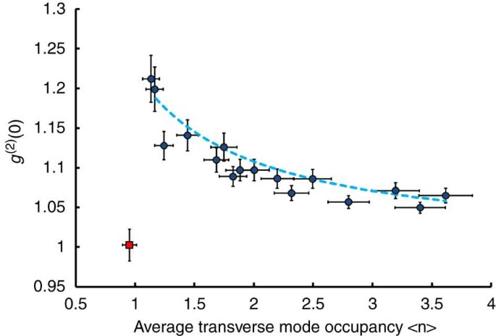Figure 5: Bunching amplitude versus mode occupancy. Graph of peak bunching amplitude as a function of average mode occupancy. A simulation of our experiment yields the theory curve shown as a dashed light blue line, in comparison with our multimode data points (blue circles). Also shown is the unity bunching amplitude when a BEC is guided (red point). Error bars in <n> indicate the uncertainty in the mode occupancy fitting procedure, whereas error bars ing(2)are due to statistical uncertainty and the normalization procedure used to calculateg(2). These are used to produce a plot of g (2) (0) against the average mode occupancy (< n >), shown in Figure 5 . Figure 5: Bunching amplitude versus mode occupancy. Graph of peak bunching amplitude as a function of average mode occupancy. A simulation of our experiment yields the theory curve shown as a dashed light blue line, in comparison with our multimode data points (blue circles). Also shown is the unity bunching amplitude when a BEC is guided (red point). Error bars in < n > indicate the uncertainty in the mode occupancy fitting procedure, whereas error bars in g (2) are due to statistical uncertainty and the normalization procedure used to calculate g (2) . Full size image A speckle pattern results from random emitters spread over a source size s , which interfere at a detector located at a distance L away from the source. The 'speckle size' is given by l=λL /2 πs , where λ is the de Broglie wavelength of the matter waves. This speckle size can be identified as the correlation length of the cloud if one identifies h/mv as the de Broglie wavelength of an atom falling at a velocity v . In our experiment, the source size is related to the transverse mode occupation of the atoms within the guide. Thus, as more transverse modes are loaded into the guide, the speckle size 'shrinks' because of the decrease in the transverse correlation length. Interestingly, as the mode occupancy decreases, the mode radius also decreases but the transverse correlation length grows making both the transverse correlation function and speckle difficult to measure. Hence, in our experiments, we measure the longitudinal/temporal correlation function and integrate over the transverse spatial dimensions. The degree of transverse coherence is then related to the bunching amplitude. In Figure 5, we plot g (2) (0) against < n > for different initial conditions. For multimode thermal guiding (blue circles), we observe an increase in bunching amplitude as the average mode occupancy decreases, due to larger transverse correlation lengths. However, when a condensate is loaded into the guide (red square), bunching vanishes, as does speckle ( Fig. 2e ), due to the presence of a single uniform wavefunction. A theoretical model of our experiment, shown as a light blue dashed line, yields reasonable agreement with our results. In conclusion, we have observed matter-wave speckle in the density distribution of guided matter waves. Analysis of the two-particle correlation function confirms that this speckle results from the same two-particle interference as demonstrated in the famous Hanbury Brown and Twiss experiment. By loading different thermal ensembles into the guide, we have been able to show that bunching increases as the average transverse mode occupancy is decreased. In the case of single-mode guiding (that is, guiding of a condensate), we observe no bunching, and no speckle, indicating that the guiding process is coherent. Finally, our experiments demonstrate that matter waves can be coherently guided (to second order) in a single mode with a near perfect gaussian spatial profile, making the guided wavefront ideal for atom interferometry. Experimental setup for producing speckle MCP images Here we use a single focused Gaussian laser beam with a 1/ e diameter of 30 μm, with maximum guiding frequencies of 1,075 and 1,500 Hz (transverse). Guiding is achieved by adiabatically ramping down the potential until the atoms escape. Experimental setup for producing g (2) correlation functions For these experiments, we use a guide with transverse frequencies of 1,700 and 2,300 Hz. Figure 4 shows the timing sequence for the experiment. Note that the guide potential is maintained constant for all the thermal runs at a value at which the BEC still remains trapped. Different thermal mode populations were then achieved by varying the depth of the initial cut. The BEC itself was guided at a slightly lower potential. Thermal distributions in the guide The thermal distributions probed via the correlation function are not in equilibrium, as, to keep the BEC trapped, the potential can only be reduced to the height of the condensate chemical potential. Thus, the low-energy tail of the thermal distribution is also still trapped. A small amount of energy is also imparted to the cloud in the transfer process. For the lowest temperatures, the guided mode consists predominately of the lowest three excited transverse modes, allowing accurate fitting of the average mode occupancy. However, for higher temperatures, < n > was scaled from the guided spot size, as there were too many modes populated to allow an accurate fit to be found. The errors shown in Figure 5 for both axes are indicative of the fitting error for the bunching amplitude and the average transverse mode occupancy. Each point on the graph in Figure 5 represents ∼ 2,000 experimental runs. Theoretical model of experiment For a perfect detector, one should measure g (2) (0)=2 for all the thermal clouds in Figure 5 . The reduction in g (2) (0) is due to binning the detection events both in time and space at the detector to provide enough correlations per bin to calculate a statistically meaningful value for g (2) (0). Transverse correlation lengths are determined by assuming free expansion of the thermal cloud once its vertical velocity is such that it is no longer adiabatically guided, combined with the transverse temperature calculated from the profile of the cloud on the detector. The associated transverse correlation length can then be calculated [24] and ranged from 200 to 370 μm. We obtained the longitudinal coherence length from fits to the temporal correlation function (such as in Fig. 3 ) for various temperatures. Convolving these lengths with the spatial and temporal bin sizes, and converting from temperature to average mode occupation by utilizing the Bose–Einstein distribution, yields the dashed theory curve in Figure 5 . How to cite this article: Dall, R. G. et al . Observation of atomic speckle and Hanbury Brown–Twiss correlations in guided matter waves. Nat. Commun. 2:291 doi: 10.1038/ncomms1292 (2011).